Flash freezing route to mesoporous polymer nanofibre networks There are increasing requirements worldwide for advanced separation materials with applications in environmental protection processes. Various mesoporous polymeric materials have been developed and they are considered as potential candidates. It is still challenging, however, to develop economically viable and durable separation materials from low-cost, mass-produced materials. Here we report the fabrication of a nanofibrous network structure from common polymers, based on a microphase separation technique from frozen polymer solutions. The resulting polymer nanofibre networks exhibit large free surface areas, exceeding 300 m 2 g −1 , as well as small pore radii as low as 1.9 nm. These mesoporous polymer materials are able to rapidly adsorb and desorb a large amount of carbon dioxide and are also capable of condensing organic vapours. Furthermore, the nanofibres made of engineering plastics with high glass transition temperatures over 200 °C exhibit surprisingly high, temperature-dependent adsorption of organic solvents from aqueous solution. The basis of the phase separation of polymer solutions is the Flory–Huggins theory proposed in 1941, since which time the technique has been widely studied [1] , [2] . The fabrication of porous polymer membranes through phase separation was intensively researched initially with regard to seawater desalination [3] . Loeb and Sourirajan, meanwhile, pioneered the preparation of asymmetric porous membranes 50 years ago by means of Dobry’s phase separation method [4] , [5] . Solvent-induced phase separation was also intensively studied as a phenomenon during the wet spinning of polymer fibres [6] , whereas the track-etching of polymer films was investigated in the early 1960s (ref. 7 ) and thermally induced phase separation was invented in the late 1970s (ref. 8 ). In the latter technique, the polymer is melted with a high boiling point solvent and then cooled. During the cooling process, the polymer and the solvent separate from one another and the resulting porous polymer is obtained after extracting the solvent. All these methods have enjoyed significant success in industrial applications. A subsequent challenge was the controlled synthesis of mesoporous polymeric materials [9] . Polymers swollen with high pressure CO 2 , for example, can form bicontinuous nanoporous materials with pores of about 40 nm when foamed by reducing the pressure at temperatures slightly below their glass transition temperatures ( T g ) (ref. 10 ). Much smaller mesopores can be induced by using inorganic porogens as templates [11] and it is also possible to form porous nanofibres by freezing polymer nanofibres prepared by electrospinning [12] , [13] . Neither process, however, has been able to produce mesoporous materials with high specific surface areas. The most elegant technique appears to be a method based on the microphase separation of block copolymers and subsequent etching, which has been actively studied since the late 1980s (refs 14 , 15 , 16 ). Mesoporous sheets obtained with block copolymers are very attractive as separation membranes [17] , [18] . Recently, Seo and Hillmyer [19] reported the formation of reticular mesoporous materials 4–8 nm in pore size using polylactide with a chain transfer agent at one terminus. This macroinitiator can polymerize a styrene/divinylbenzene mixture and the resulting copolymer induces a phase separation structure. These new techniques have enabled the preparation of mesoporous polymeric materials with narrow pore size distributions. Nevertheless, solvent-induced and thermally induced phase separation methods have long been used in industries as they are considered the simplest and most well-established methods of producing porous polymer architectures, as they are tunable to many different polymers and applications. The key factors affecting the pore formation mechanism include phase separation of the solvent, gelation of the polymer solution and crystallization of the polymers [20] , [21] . Freeze drying of polymer solutions has also been examined as a means of controlling porous structure [22] , but it remains very challenging to fabricate mesoporous materials through the phase separation of common polymers. The major difficulty is in controlling the long-range diffusion of solvent molecules, which causes undesirable coarsening of the solvent-rich phase. To restrict solvent diffusion to the nanometre range, we carefully examined a phase separation system operating under deep frozen conditions. Herein, we report that the crystallization of solvent molecules far below their freezing point temperature results in extremely fine microphase separation and that an interconnected polymer nanofibre network may be formed by subsequently extracting the solvent molecules at low temperature. Concept of flash freezing route During fabrication of the mesoporous polymer ( Fig. 1a ), a concentrated polymer solution (10–40 wt%) is first frozen using liquid nitrogen (−196 °C). The solvent molecules subsequently transition to a glassy state between the entangled polymer chains. In the second step, the temperature is slowly increased to produce cold crystallization of the frozen solvent molecules. During this crystallization, the polymer chains are expelled from solvent nanocrystals, producing a nanofibre network structure, which effectively suppresses further growth of the solvent nanocrystals. Finally, extracting the nanocrystallized solvent using a poor solvent at low temperature yields a highly porous nanofibre network. 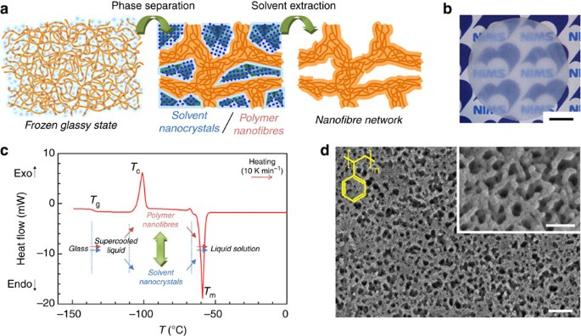Figure 1: Fabrication of nanofibre networks. (a) Formation mechanism of a polymer nanofibre network through solvent nanocrystallization. (b) Photograph of disk-shaped PSF sheet (mould dimensions: 25 × 1 mm, thickness: 0.7–0.8 mm, scale bar, 5 mm). (c) DSC plot of a 20 wt% PS solution in DMF (heating rate: 10 K min−1). (d) SEM image of a PS nanofibre network and enlarged image (inset), showing the highly porous structure formed after removal of nanocrystallized DMF (NF2 inTable 1). Scale bar, 250 nm (inset: 100 nm). The sample was prepared from 20 wt% DMF solution. Figure 1: Fabrication of nanofibre networks. ( a ) Formation mechanism of a polymer nanofibre network through solvent nanocrystallization. ( b ) Photograph of disk-shaped PSF sheet (mould dimensions: 25 × 1 mm, thickness: 0.7–0.8 mm, scale bar, 5 mm). ( c ) DSC plot of a 20 wt% PS solution in DMF (heating rate: 10 K min −1 ). ( d ) SEM image of a PS nanofibre network and enlarged image (inset), showing the highly porous structure formed after removal of nanocrystallized DMF (NF2 in Table 1 ). Scale bar, 250 nm (inset: 100 nm). The sample was prepared from 20 wt% DMF solution. Full size image Macroporous polymers can be prepared by crystallizing solvents from the liquid state, then the growth of large crystals causes the frozen solution to take on a white, opaque appearance [23] . In contrast, the rapid freezing in liquid nitrogen used in our process generates transparent frozen solutions, indicating that macrocrystals are not formed over the entire sample. Differential scanning calorimetry (DSC) additionally revealed that the solvent glassified during cooling ( Supplementary Fig. S1 ). To quantitatively evaluate the cold crystallization of solvents, we performed DSC measurements at elevated temperatures. As its temperature is increased, the DSC curve of a frozen dimethylformamide (DMF) solution of 20 wt% polystyrene (PS) ( Fig. 1c ) shows a baseline shift at −136 °C, followed by an exothermic peak ( T c ) at −105 °C and an endothermic peak ( T m ) at −61 °C. The baseline shift indicates a transition of the solvent from the glassy state to an extremely supercooled liquid (or a more liquid-like glass) state, while the two peaks demonstrate that cold crystallization of DMF and melting of the nanocrystals occur. The enthalpy associated with cold crystallization ( H c , 57.0 J g −1 ) was similar to that of melting ( H m , 56.0 J g −1 ), indicating that all the solvent molecules crystallized at the elevated temperature. The observed enthalpy of melting ( H m ) of DMF nanocrystals in a PS nanofibre network was 83% that of pure DMF crystals reported in the database [24] . Mesoporous PS nanofibres were obtained after extracting the nanocrystallized solvent with methanol at −80 °C. Scanning electron microscopy (SEM) cross sections revealed a uniform fibrous morphology free of macrovoids ( Fig. 1d ). As seen in the high magnification image, the specimens consist of highly branched nanofibres connected with one another. The diameter distribution of the nanofibres was analysed based on more than 1,000 points in SEM images ( Supplementary Figs S2 and S3 ), and then Gaussian fitting gave an average diameter of 17.6±5.6 nm, assuming that the nanofibres have circular cross sections. Mesoporous structure was much finer when PS concentration was 40 wt% ( Supplementary Fig. S2 ). The Brunauer–Emmett–Teller (BET) model was used for the analysis of nitrogen adsorption isotherms at low pressures ( p / p 0 <0.3). The specific surface area ( S BET ) of PS nanofibre network obtained from 40 wt% DMF solution was found to be 196 m 2 g −1 with maximum adsorption as high as 432 cm 3 STP g −1 at pressure approaching saturation ( p / p 0 =0.99), indicating that the interconnected open mesopores allow rapid nitrogen diffusion into the inner regions of the sample. The Barrett–Joyner–Halenda (BJH) model, which employs the Young–Laplace equation for capillary condensation of nitrogen, was used to determine the pore size distribution from the isotherm at higher pressures ( p / p 0 >0.3) ( Supplementary Fig. S4 ). The pore volumes of mesopores (radius: 1–25 nm) and macropores (radius: 25–100 nm) were calculated to be 0.66 and 0.01 cm 3 g −1 , respectively. Phase separation in the frozen state was applied to various polymers, as summarized in Table 1 . These polymers produced average nanofibre diameters in the range of 12–21 nm. Polysulfone (PSF) nanofibres had an average diameter of 14.2 nm along with S BET value of 264 m 2 g −1 , whereas poly(vinyl chloride) (PVC) nanofibres had the thickest diameter (20.7 nm) and the lowest S BET value of 124 m 2 g −1 . The geometric specific surface areas ( S calc ) of these materials are consistent with the corresponding S BET values within a difference of 30%, indicating that the specific surface area is primarily due to the free surface of the nanofibres. Pore size distributions calculated from sorption isotherms were narrow and the average radius obtained from the desorption process ( r D ) was significantly smaller than that measured using the adsorption process ( r A ), as often seen in capillary condensation of nitrogen in mesopores [15] . An approximate value of the bifurcation density of the nanofibres could be estimated from these parameters. For example, the average distance between adjacent PSF nanofibre junctions was 31 nm, as calculated from the pore radius of 8.5 nm and the nanofibre diameter of 14.2 nm. PS had the largest total pore volume (1.44 cm 3 g −1 ), whereas PSF, poly(bisphenol-A-carbonate) (PC), poly( p -phenylene ether-sulfone) (PES) and polyacrylonitrile (PAN) had mesopore volumes in the range of 0.80–0.93 cm 3 g −1 . Figure 1b shows a photograph of a disk-shaped sheet prepared from 20 wt% DMF solution of PSF. The bulk density was as low as 0.318 g cm −3 . When a PSF sheet produced in this form was placed into a glass vial filled with ethanol, it was observed to rapidly absorb ethanol and sink to the bottom of the vial, as the sheet has a percolating network of mesopores from one side to the other. The actual density of the PSF nanofibres was determined using a helium pycnometer to be 1.25±0.04 g cm −3 , which is almost equal to that of the corresponding bulk polymer. The internal morphology of the nanofibre network was confirmed by obtaining 3D tomography images via transmission electron microscopy ( Supplementary Fig. S5 , Supplementary Movie 1 and Supplementary Methods ). Table 1 Structural properties of polymer nanofibre networks. Full size table Control of mesoporous structure A key factor in creating a mesoporous structure is attaining cold crystallization near T g . When a polymer solution is slowly cooled, the solvent crystallizes at a temperature slightly below its melting point ( T m ). Conversely, flash freezing vitrifies the solution without allowing solvent crystallization ( Supplementary Fig. S1 ). When the temperature is then slowly increased, cold crystallization (essentially phase separation in the frozen state) is initiated. This crystallization process, however, results in an increase of the polymer concentration within the polymer-rich phase, such that the polymer concentration approaches the green T g line in Fig. 2a , and further solvent crystallization is then restricted by the glassy polymer-rich phase. Experimental values obtained for the PS/ o -xylene system are plotted in Fig. 2b , where T f (solvent crystallization temperature) and T g were obtained from cooling DSC thermograms (−70 K min −1 ) and T c and T m were obtained from heating thermograms (10 K min −1 ). Over the initial polymer concentration range of 30–60 wt% (range [1] in Fig. 2b ), only mesopores are produced. In contrast, macropores are also generated in range [2]. The total pore volume ( V total ) was observed to increase with decreasing PS concentration, although the maximum value of mesopore volume ( V meso ) was obtained near 20 wt% ( Fig. 2c ). The mesopore volumes obtained were significantly different when employing each of the three isomers of xylene. In the case of m -xylene ( T m : −48 °C) the formation range of mesopores (range [1]) was shifted to lower PS concentrations and the V meso value was more than 1.5 cm 3 g −1 even in a 10 wt% PS solution. In sharp contrast, p -xylene ( T m : 13 °C) produced a very small V meso value at a PS concentration below 40 wt%. This occurs because range [1] shifts to higher PS concentrations when T m and T c are high. It is also known that p -xylene has no tendency to transition to the glassy state at experimentally obtainable cooling rates [25] , indicating that this solvent readily forms macrocrystals. 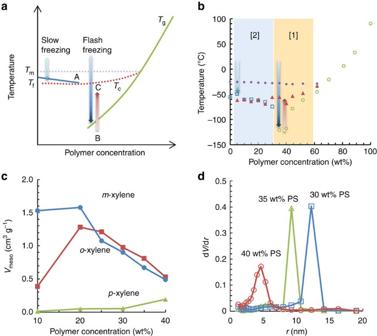Figure 2: Binary phase diagram and pore size distributions. (a) Binary phase diagram of the polymer/solvent system.Tg, glass transition temperature of polymer (green line);Tm, solvent melting point (purple dotted line);Tf, solvent crystallization temperature (blue line);Tc, solvent cold-crystallization temperature (red dotted line). (b) Phase diagram of the PS/o-xylene system. Open circles,Tg; solid diamonds,Tm; open squares,Tf; solid triangles,Tc. (c) Mesopore volumes of PS nanofibre networks prepared fromm-xylene (blue),o-xylene (red) andp-xylene (green) solutions. (d) Pore size distributions of PS nanofibre networks fabricated from 40 wt% (red), 35 wt% (green) and 30 wt% (blue)m-xylene solutions. Figure 2: Binary phase diagram and pore size distributions. ( a ) Binary phase diagram of the polymer/solvent system. T g , glass transition temperature of polymer (green line); T m , solvent melting point (purple dotted line); T f , solvent crystallization temperature (blue line); T c , solvent cold-crystallization temperature (red dotted line). ( b ) Phase diagram of the PS/ o -xylene system. Open circles, T g ; solid diamonds, T m ; open squares, T f ; solid triangles, T c . ( c ) Mesopore volumes of PS nanofibre networks prepared from m -xylene (blue), o -xylene (red) and p -xylene (green) solutions. ( d ) Pore size distributions of PS nanofibre networks fabricated from 40 wt% (red), 35 wt% (green) and 30 wt% (blue) m -xylene solutions. Full size image Regardless of the types of solvent, solvent crystallization at point A in Fig. 2a always results in the formation of several micrometer-sized pores and thus, to ensure the selective formation of mesopores, the polymer solution should be rapidly cooled to below the T g line (at point B). Cold crystallization in the frozen state is very slow, and so the solution temperature must be maintained below the melting point of the solvent (point C) for several hours. We have found that, over certain ranges of concentration and temperature, bicontinuous mesoporous structures composed of polymer nanofibres will form. This finding may be the most important extension of the basic principles of thermally induced phase separation since Castro proposed the process in the late 1970s (ref. 8 ). The mesopores decrease in size with increasing concentrations of the polymer solution, likely due to the strong steric inhibition effect of the nanofibre network. Figure 2d shows the results obtained from a PS/ m -xylene system. Based on pore size distributions calculated from the BJH model, the pore radii were 12.2, 9.2 and 4.7 nm in the materials obtained from 30, 35 and 40 wt% PS solutions, respectively. The pore radii obtained from the desorption isotherms were much smaller, giving values of 6.9 and 2.7 nm for the mesoporous materials from 30 and 40 wt% PS solutions. In general, mesopores smaller than 5 nm in radius readily collapse under the effects of the strong Laplace force [19] and therefore we believe that pores of radius 2.7 nm are the smallest which PS, with a T g of ~100 °C, can achieve. Materials properties and processing The thermal stability of our mesoporous polymer nanofibre networks was confirmed by temperature-modulated differential scanning calorimetry (MDSC) measurements. All samples exhibited their primary T g at the same temperature as the bulk polymer although we observed a minor change in specific heat capacity at temperatures 20–30 °C below the primary T g ( Supplementary Fig. S6 ). We can conclude that the PSF nanofibres are thermally stable up to 150 °C ( Supplementary Table S3 ), although their mechanical properties are evidently impacted by their significant porosity (56%). As an example, the Young’s modulus measured for the mesoporous PSF sheets was 0.23±0.02 GPa ( Supplementary Fig. S7 ), which is less than the elastic modulus of bulk PSF (2.5–2.6 GPa) [26] . The stress at break ( σ b ) and the elongation of the nanofibre network were 7.4±0.6 MPa and 26.5±9.0%, respectively. The former value is approximately one-tenth that of non-porous PSF ( σ b : 70 MPa). These polymer nanofibre networks can be obtained in the form of large sheets, fibres and pellets ( Fig. 3a–c ); the extrusion of PS solution into a cooled coagulation bath (methanol at −100 °C), for example, produced macroscopic fibres composed of polymer nanofibres. The mass-produced fibres also exhibit extremely high specific surface areas, as high as 328 m 2 g −1 . To the best of our knowledge, this is the highest surface area value reported to date for conventional glassy polymers. These fibres were subsequently cut into pellets with a mechanical crusher and used for separation experiments. It was also possible to tune the appearance of macro and mesopores by controlling both the polymer concentration and solvent crystallization conditions ( Supplementary Fig. S8 ). 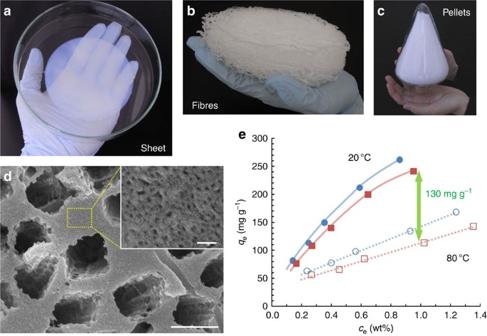Figure 3: Macro- and microscopic morphology control and temperature dependent adsorption. (a) Large sheet form PSF nanofibre network (thickness: 45 μm) obtained from 20 wt% N-methyl-2-pyrrolidone solution. (b) Fibre form PS nanofibre network (SBET: 328 m2g−1,Vmeso: 0.72 cm3g−1andVmacro: <0.01 cm3g−1). (c) Pellet form PS nanofibre network. Fibre and pellet forms were obtained from 40 wt% DMF solutions. (d) SEM cross-section of macroporous material made of mesoporous PS nanofibre network prepared from 30 wt% DMAc solution (SBET: 144 m2g−1,Vmeso: 0.33 cm3g−1andVmacro: 0.22 cm3g−1). Inset indis an enlarged image of the region in the yellow box. Scale bar, 500 nm (inset: 50 nm). (e) Adsorption isotherms ofm-cresol dissolved in pure water. Blue circles: PES nanofibre network. Red squares: PSF nanofibre network. Solid and open symbols represent the adsorption at 20 °C and 80 °C, respectively. Figure 3d shows cross-sectional SEM images of a PS nanofibre network produced from a 30 wt% dimethylacetamide (DMAc) solution using liquid nitrogen. Similarly to the range [2] of PS/ o -xylene system ( Fig. 2b ), both macropores and mesopores form at this concentration. The inclusion of macropores significantly improves the accessibility of adsorbate molecules to mesopores. Thermally stable engineering plastics may form extremely small pores. For example, a polyetherimide nanofibre network ( T g : 217 °C) prepared from the mixed solution of dimethylsulfoxide and DMAc have a S BET value of 301 m 2 g −1 and a narrow mesopore radius distribution near 1.9 nm ( Supplementary Fig. S9 ), which is the smallest value experimentally obtained for mesoporous polymeric materials [19] . Figure 3: Macro- and microscopic morphology control and temperature dependent adsorption. ( a ) Large sheet form PSF nanofibre network (thickness: 45 μm) obtained from 20 wt% N-methyl-2-pyrrolidone solution. ( b ) Fibre form PS nanofibre network ( S BET : 328 m 2 g −1 , V meso : 0.72 cm 3 g −1 and V macro : <0.01 cm 3 g −1 ). ( c ) Pellet form PS nanofibre network. Fibre and pellet forms were obtained from 40 wt% DMF solutions. ( d ) SEM cross-section of macroporous material made of mesoporous PS nanofibre network prepared from 30 wt% DMAc solution ( S BET : 144 m 2 g −1 , V meso : 0.33 cm 3 g −1 and V macro : 0.22 cm 3 g −1 ). Inset in d is an enlarged image of the region in the yellow box. Scale bar, 500 nm (inset: 50 nm). ( e ) Adsorption isotherms of m -cresol dissolved in pure water. Blue circles: PES nanofibre network. Red squares: PSF nanofibre network. Solid and open symbols represent the adsorption at 20 °C and 80 °C, respectively. Full size image Flash freezing route appears to be very close to the freeze-drying method that is commonly used to make tissue engineering scaffolds [13] . However, the conventional method has some practical difficulties. To form solvent nanocrystals, good solvent needs to have crystallization temperature near T g of polymer solution, which usually appears at low temperature. However, the nanocrystals formed at low temperature are very hard to be removed via vacuum process. On the other hand, the solvents with relatively high crystallization temperature, for example, p -xylene can be readily removed via vacuum process. Note that sublimation rate becomes high with increasing melting temperature. However, such solvents cannot form the nanocrystals at experimentally achievable cooling rate. The advantage of solvent extraction in flash freezing route is that the extraction rate is high even at −80 °C. Because of the high values of free surface area and percolating pores, these materials exhibited a variety of interesting separation properties. Mesoporous PSF sheets could be used for ultrafiltration of 5 nm nanoparticles with a rejection rate above 90% ( Supplementary Table S4 ). The nanofibre networks were also able to rapidly adsorb CO 2 and the Henry’s constant was about three times larger than that of the bulk polymer ( Supplementary Figs S10 and S11 and Supplementary Table S5 ) [27] , [28] . Condensation of organic vapours into the mesopores was also found to be extremely sensitive to pressure and temperature ( Supplementary Fig. S12 ) [29] . The most important is the fact that mesoporous polymers are capable of separating toluene from aqueous solutions a few tens of ppm in concentration and can also adsorb a significant amount of tetrahydrofuran from aqueous solution ( Supplementary Fig. S13 ). The adsorption isotherms of m -cresol are shown in Fig. 3e . By choosing PES, an engineering plastic with a very high T g value near 225 °C, we were able to generate thermally stable mesoporous pellets with very high adsorption capacities up to 262 mg g −1 ( Supplementary Table S6 ). From a practical point of view, it is important that the adsorption abilities of PES and PSF nanofibres are very sensitive to ambient temperature. The difference in the values at 20 and 80 °C (130 mg g −1 at m -cresol concentration of 1.0 wt%) was more than two times greater than the best values obtained for commercially available activated carbons and cross-linked polymer adsorbents in our comparison experiments ( Supplementary Fig. S14 ). In principle, temperature-sensitive adsorbents can be reactivated by circulating steam from the boiler. We believe that our mesoporous polymer adsorbents will contribute to the purification of industrial drainage and so-called produced water from oil and gas fields [30] . A bench-scale separator unit incorporating these reusable oil adsorbents is currently being studied in our laboratory. Fabrication procedures Detailed information of polymers (supplier, molecular weight, actual density, T g , T m and price) and the fabrication conditions for the nanofibre network (solvent, polymer concentration and solvent extraction procedures) are described in Supplementary Tables S1 and S2 and Supplementary Note 1 . Disk-shaped nanofibre sheets were fabricated using a ring-shaped Teflon mould (inner diameter: 25 mm; thickness: 1 mm) placed between two copper plates covered with a 0.05-mm-thick Teflon film. The polymer solution was frozen by immersing the mould in liquid nitrogen. Large sheets of polymer nanofibre networks were prepared by a simple spin-coating technique, in which the polymer solution was first spread on a glass plate of 100 mm in diameter and then immediately immersed in excess methanol precooled to −100 °C. Macroscopic fibres of polymer nanofibre networks were prepared by directly injecting the polymer solution into excess methanol precooled to −100 °C, using a metal syringe with a needle with a 0.5 mm inner diameter ( Supplementary Movie 2 ). The extraction was performed for one day in a cryogenic freezer (−80 °C), following which residual methanol in the solidified sample was exchanged with tert-butanol at room temperature and the sample was freeze dried ( Supplementary Methods ). DSC measurements The freezing and melting behaviours of a polymer solution were characterized by DSC (TA Instruments, Q2000), which was also used for the determination of T g line shown in Fig. 2b . MDSC measurements were performed using the Q2000 with a temperature amplitude of ±1 K and 60 s cycle at a constant heating rate of 2 K min −1 . Details of each measurement are described in the Supplementary Figs S1, S6 and S8 and Supplementary Methods . SEM observations The morphologies of the polymer nanofibre networks were observed by field-emission SEM (Hitachi, FE-SEM S-4800). Sample preparation was accomplished by immersing a sheet of the nanofibre network in ethanol followed by freeze fracturing in liquid nitrogen ( Supplementary Methods ). A cross-section of the specimen was attached to an SEM sample holder by carbon adhesive tape and a 1.5-nm-thick platinum layer was deposited by ion sputtering (Hitachi, E-1030) at an argon pressure of 7 Pa and a current density of 10 mA for 30–60 s to prevent electric charging during SEM observations. The deposition thickness was monitored using a quartz crystal microbalance. Gas adsorption measurements Nitrogen adsorption isotherms at 77 K were measured using a volumetric gas adsorption apparatus (BEL Japan, Belsorp-max). A glass sample tube was filled with small pieces of dried sample (40–70 mg) and thoroughly dried in vacuum at 70 °C overnight (except for PVC, which was dried at 50 °C). All the measurements were performed after conducting a 3-min leak check to ensure sufficient sealing and complete drying of the specimens. BET and BJH analyses were systematically performed using commercially available software (BEL Japan, BEL Master). CO 2 sorption isotherms up to 30 atm were measured using a volumetric gas sorption system (BEL Japan, Belsorp-HP). As CO 2 gas shows no-ideal behaviour at high pressure, the sorption data were corrected using virial coefficient at each temperature, considering the volume of the polymer nanofibre network in the cell and very slight baseline changes due to the sorption to the empty cell. The sorption isotherms were analysed using the dual-mode sorption model to determine the Henry’s constant ( Supplementary Methods ). Adsorption of m -cresol The concentrations of m -cresol in Fig. 3e are in the range of 0.51–2.04 wt%. During adsorption experiments, the aqueous solution of m -cresol (20.0 g) and a sample of mesoporous polymer (0.9 g) were placed in a 20 ml glass vial and sealed with a PTFE (polytetrafluoroethylene)-coated butyl rubber/aluminium septum (La-Pha-Pack). Equilibrium was confirmed by repeatedly monitoring the adsorption amount over a period of 24–72 h. At set time intervals, the concentration of m -cresol in the aqueous phase was measured using gas chromatography (Shimadzu, GC-2014) employing N 2 as the carrier gas. The measurement system also included a hydrogen flame ionization detector and a PerkinElmer headspace sampler (TurboMatrix, HS40). In order to correct for the effects of evaporation (usually <3%), m -cresol solutions without added mesoporous polymer nanofibre networks were also examined, and the results were used as blanks. The adsorption amount of m -cresol ( q e , in mg g −1 ) was calculated using the following equation: where C i is the concentration of the blank (wt%), C e is the concentration under equilibrium conditions (wt%), W s is the weight of solution (g) and W p is the weight of adsorbent (g). How to cite this article: Samitsu, S. et al . Flash freezing route to mesoporous polymer nanofibre networks. Nat. Commun. 4:2653 doi: 10.1038/ncomms3653 (2013).